SIRT6 is required for maintenance of telomere position effect in human cells In Saccharomyces cerevisiae , the repressive chromatin environment at telomeres gives rise to telomere position effect (TPE), the epigenetic silencing of telomere-proximal genes. Chromatin-modifying factors that control TPE in yeast have been extensively studied, and, among these, the lifespan regulator and silencing protein Sir2 has a pivotal role. In contrast, the factors that generate and maintain silent telomeric chromatin in human cells remain largely unknown. Here we show that the Sir2 family member SIRT6 is required for maintenance of TPE in human cells. RNAi-mediated depletion of SIRT6 abrogates silencing of both an integrated telomeric transgene and an endogenous telomere-proximal gene. Moreover, enhanced telomeric silencing in response to telomere elongation is associated with increased repressive chromatin marks, and this heterochromatic milieu is lost in SIRT6-deficient cells. Together, these findings establish a new role for SIRT6 in regulating an ageing-associated epigenetic silencing process and provide new mechanistic insight into chromatin silencing at telomeres. In Saccharomyces cerevisiae , the NAD + -dependent histone deacetylase Sir2 (silent information regulator 2) has a key role in generating and maintaining silent chromatin near telomeres. This epigenetic silencing of telomere-proximal genes—a phenomenon termed telomere position effect (TPE) [1] , [2] , [3] , [4] —is lost with replicative yeast ageing, concomitant with aberrant hyperacetylation of sub-telomeric histones [5] , [6] . One important feature of TPE is that the strength of silencing increases with telomere length [7] , [8] , a property thought to reflect an increased repressive chromatin environment that results from longer telomeres [9] , [10] . Like their yeast counterparts, mammalian telomeres can exert silencing effects on adjacent genes [11] , [12] , [13] . However, aside from downstream changes, such as altered histone methylation patterns and suggestions that HP1 is involved [12] , [14] , the upstream factors required for telomeric gene silencing in human cells remain largely unknown. The Sir2-family member SIRT6 is a highly substrate-specific histone deacetylase that promotes proper chromatin function in several physiologic contexts, including genome stabilization, DNA repair, and gene expression. Early work implicated SIRT6 in regulating ageing-associated pathologies and lifespan in mice [15] . Subsequently, SIRT6 was shown to possess NAD + -dependent histone deacetylase activity, with specificity for lysines 9 and 56 of histone H3 (H3K9 and H3K56, respectively) [16] , [17] , [18] . Since the discovery of its enzymatic activity, SIRT6 has been shown to function in several important genomic contexts. First, SIRT6 modulates telomeric chromatin in mammalian cells [16] , [17] . By deacetylating H3K9 and H3K56 at telomeres during S-phase, SIRT6 is required for proper replication of telomeres. Depletion of SIRT6 from human cells results in abnormal telomere structures and stochastic replication-associated telomere sequence loss, ultimately leading to genomic instability, chromosomal end-to-end-fusions, and premature cellular senescence [11] . In addition to its role at telomeres, SIRT6 also has a critical role in regulating DNA repair. SIRT6 associates dynamically with chromatin flanking DNA double-strand breaks and is required for stabilization of the non-homologous end-joining protein DNA-PKcs at double-strand breaks and for efficient repair of these breaks [19] . Recently, SIRT6 was shown to promote DNA double-strand break repair through several further mechanisms, including stimulating DNA end-resection in homology-directed repair [20] and activating the poly-ADP ribosyltransferase PARP-1 to promote non-homologous end-joining and homology-directed repair [21] . Finally, histone deacetylation by SIRT6 is important for active transcriptional repression of gene expression networks linked to ageing and metabolism [22] , [23] . For example, SIRT6 functions at specific NF-κB target gene promoters to attenuate gene expression, providing an important link between SIRT6 and active gene repression [22] . More recently, SIRT6 was also shown to repress expression of genes involved in glucose and fat metabolism [23] , [24] , [25] , [26] . However, no role for SIRT6 in the generation or maintenance of silent chromatin domains—at telomeres or elsewhere—has yet been described. Here we uncover a new role for SIRT6 in maintaining TPE in human cells. We show that SIRT6 dynamically regulates the silencing of a telomere-proximal transgene and that depletion of SIRT6 leads to loss of TPE-associated heterochromatic marks. In addition, we show that SIRT6 is required for the repression of an endogenous telomere-proximal gene. These findings indicate that SIRT6 is important for maintaining a proper telomeric chromatin structure that is required for silencing of nearby genes. Silencing of a telomere-proximal reporter gene requires SIRT6 The growing evidence that proper chromatin silencing is important for mammalian ageing and cancer, together with the site-specific histone deacetylation activity and telomeric functions of SIRT6, led us to ask whether SIRT6 modulates TPE in human cells. To address this question, we used a previously established luciferase-based system that recapitulates important features of TPE in yeast. In this system, a luciferase reporter gene is stably integrated into the genome of human cervical cancer (HeLa) cells at either a telomeric position or an internal chromosomal position ( Fig. 1a , ref 11 ). As previously shown, overexpression of human telomerase reverse transcriptase (hTERT) in these cells—and concomitant lengthening of bulk telomeres—dramatically reduced telomeric luciferase expression ( Fig. 1b , ref 11 ), indicating that the strength of silencing is proportional to telomere length, as has been observed in yeast [7] , [8] . These data confirm that our system recapitulates important features of the Sir2-dependent silencing of telomere-proximal genes in yeast. 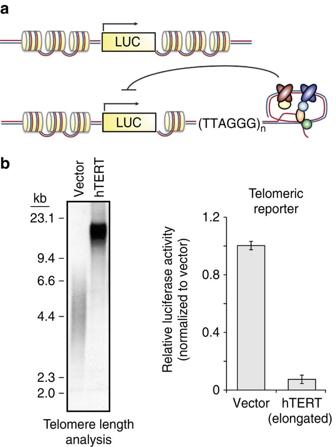Figure 1: Cell-based system for studying TPE in human cells. (a) Schematic of the HeLa luciferase TPE model system11, depicting internal (top) and telomeric (bottom) reporters. Inhibitory arrow represents silencing effect of repressive chromatin at telomeres. (b) Effect of ectopic hTERT on expression of telomeric luciferase. Left: Telomere length (in kilobasepairs (kb)) was determined by terminal restriction fragment analysis. Right: Average luciferase expression from three independent siRNA transfections; error bars represent ±s.d. Figure 1: Cell-based system for studying TPE in human cells. ( a ) Schematic of the HeLa luciferase TPE model system [11] , depicting internal (top) and telomeric (bottom) reporters. Inhibitory arrow represents silencing effect of repressive chromatin at telomeres. ( b ) Effect of ectopic hTERT on expression of telomeric luciferase. Left: Telomere length (in kilobasepairs (kb)) was determined by terminal restriction fragment analysis. Right: Average luciferase expression from three independent siRNA transfections; error bars represent ±s.d. Full size image We next used this system to ask whether SIRT6 is required for TPE in human cells. Small interfering RNA (siRNA)-mediated depletion of SIRT6 significantly increased telomeric luciferase expression, and this effect was particularly strong in cells with long telomeres ( Fig. 2a ). In contrast, SIRT6 depletion did not affect the expression of an internally integrated luciferase gene, highlighting the specificity of the de-repression ( Fig. 2a ). This telomere-specific loss of silencing was also observed in a second set of cell lines in which the luciferase genes were integrated at distinct telomeric and internal sites ( Fig. 2b ); we note that the differential effect of SIRT6 depletion on telomeric luciferase expression in the two cell lines is consistent with observed differences in the repressive capacity of different telomeres in yeast [27] . A second independent SIRT6-directed siRNA revealed a dose-dependent effect of SIRT6 depletion on loss of telomeric silencing ( Fig. 2c,e ). In contrast, depletion of SIRT1—another nuclear Sir2 family member recently linked to telomere function [28] —did not trigger telomere-specific de-repression but instead had a rather subtle effect on both telomeric and non-telomeric luciferase expression ( Fig. 2d ). Together, these observations reveal that SIRT6 is specifically required for maintaining efficient TPE in human cells. 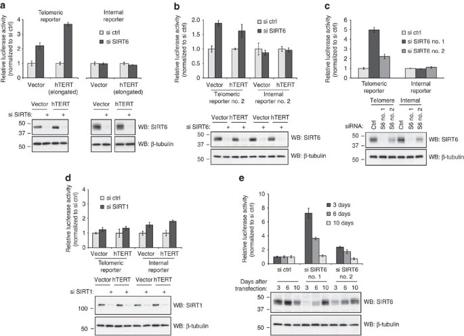Figure 2: Effect of SIRT6 depletion on expression of a telomeric luciferase transgene. (a) Relative luciferase activity in cells harbouring a telomeric (left) or internal (right) luciferase transgene, transfected with control siRNA or siRNA targeting SIRT6. Cells were collected for luciferase assays∼72 h after siRNA transfection. (b) Relative luciferase activity in a second independent set of telomeric and internal luciferase cell lines, transfected with SIRT6-directed siRNA and collected as in (a). (c) Relative luciferase activity in cells transfected with control siRNA or two independent SIRT6 siRNAs, collected as in (a). (d) Relative luciferase activity in cells transfected with control siRNA or siRNA targeting SIRT1 and collected as in (a,c). Fora–d, luciferase activity is normalized to control siRNA-transfected cells; results are from three independent siRNA transfections; error bars represent ±s.d. (e) Telomeric luciferase cells expressing ectopic hTERT were transfected with the indicated siRNAs, and luciferase assays were performed at the indicated time-points after transfection. Luciferase activity is normalized to control siRNA-transfected cells at each time-point; results are from three independent siRNA transfections; error bars represent ±s.d. Figure 2: Effect of SIRT6 depletion on expression of a telomeric luciferase transgene. ( a ) Relative luciferase activity in cells harbouring a telomeric (left) or internal (right) luciferase transgene, transfected with control siRNA or siRNA targeting SIRT6. Cells were collected for luciferase assays ∼ 72 h after siRNA transfection. ( b ) Relative luciferase activity in a second independent set of telomeric and internal luciferase cell lines, transfected with SIRT6-directed siRNA and collected as in ( a ). ( c ) Relative luciferase activity in cells transfected with control siRNA or two independent SIRT6 siRNAs, collected as in ( a ). ( d ) Relative luciferase activity in cells transfected with control siRNA or siRNA targeting SIRT1 and collected as in ( a , c ). For a – d , luciferase activity is normalized to control siRNA-transfected cells; results are from three independent siRNA transfections; error bars represent ±s.d. ( e ) Telomeric luciferase cells expressing ectopic hTERT were transfected with the indicated siRNAs, and luciferase assays were performed at the indicated time-points after transfection. Luciferase activity is normalized to control siRNA-transfected cells at each time-point; results are from three independent siRNA transfections; error bars represent ±s.d. Full size image Many chromatin modifications are highly dynamic, as evidenced by the reversibility of TPE in yeast [1] . To determine whether the loss of telomeric luciferase silencing in SIRT6-depleted cells is reversible, we transiently transfected cells with SIRT6-directed siRNAs and collected the cells at various time-points after transfection. Recovery of SIRT6 expression over time was sufficient to re-establish silencing of the telomeric luciferase gene ( Fig. 2e ), indicating that SIRT6 dynamically regulates TPE. This reversibility also argues that the observed changes in luciferase expression result directly from epigenetic effects on chromatin silencing, and not from any irreversible gross chromosomal abnormalities that have been observed in cells stably depleted of SIRT6 (ref. 16 ). Indeed, neither telomere dysfunction nor telomere sequence loss was elevated during the short time-frame of the transient SIRT6 knockdown in our experiments ( Fig. 3 ), indicating that SIRT6 influences telomeric gene silencing via a mechanism that is independent of such abnormalities. 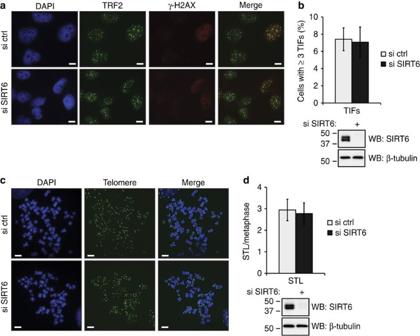Figure 3: Analysis of telomere dysfunction and chromosomal integrity in response to transient SIRT6 knockdown. (a) Representative images of control and SIRT6-depleted telomeric luciferase HeLa cells stained with antibodies against TRF2 (green) and γ-H2AX (red). Scale bars, 10 μm. (b) Quantification of telomere dysfunction-induced foci (TIFs) from (a). TIFs were detected by co-localization of TRF2 and γ-H2AX, and cells with at least 3 TIFs were scored. Data represent averages of 3–6 fields (10–30 cells per field), ±s.e.m.P=0.905, two-tailed Student'st-test. (c) Representative telomere FISH images of metaphase spreads from control and SIRT6-depleted telomeric luciferase HeLa cells. Scale bars, 10 μm. (d) Quantification of sister telomere loss (STL) from (c). Signal-free ends were scored. Data represent averages of 18 metaphases, ±s.e.m.P=0.815, two-tailed Student'st-test. Figure 3: Analysis of telomere dysfunction and chromosomal integrity in response to transient SIRT6 knockdown. ( a ) Representative images of control and SIRT6-depleted telomeric luciferase HeLa cells stained with antibodies against TRF2 (green) and γ-H2AX (red). Scale bars, 10 μm. ( b ) Quantification of telomere dysfunction-induced foci (TIFs) from ( a ). TIFs were detected by co-localization of TRF2 and γ-H2AX, and cells with at least 3 TIFs were scored. Data represent averages of 3–6 fields (10–30 cells per field), ±s.e.m. P =0.905, two-tailed Student's t -test. ( c ) Representative telomere FISH images of metaphase spreads from control and SIRT6-depleted telomeric luciferase HeLa cells. Scale bars, 10 μm. ( d ) Quantification of sister telomere loss (STL) from ( c ). Signal-free ends were scored. Data represent averages of 18 metaphases, ±s.e.m. P =0.815, two-tailed Student's t -test. Full size image Maintenance of TPE-associated heterochromatic marks requires SIRT6 To examine the underlying chromatin changes involved in TPE in human cells, we used chromatin immunoprecipitation (ChIP) to measure the occupancy of total histone H3, histone H3 acetylated at lysine 9 (H3K9Ac, a marker of transcriptionally active chromatin), and histone H3 tri-methylated at lysine 9 (H3K9me3, a marker of constitutive heterochromatin) at several loci within the telomeric luciferase gene ( Fig. 4a ). 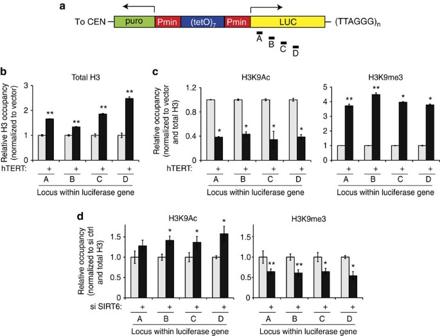Figure 4: Characterization of telomere-proximal chromatin changes triggered by telomere elongation and SIRT6 depletion. (a) Schematic of the luciferase cassette and real-time PCR primers used in ChIP experiments inb–d. The palindromic nature of the promoter region of the integrated luciferase plasmid precluded the use of primers upstream of the luciferase gene. CEN, centromere. (b) Analysis of total H3 occupancy within the telomeric luciferase gene in response to telomere elongation. Data are representative of at least two independent experiments. Light grey bars, vector-transduced cells; dark grey bars, hTERT-transduced cells. (c) Analysis of histone marks within the telomeric luciferase gene in response to telomere elongation. Occupancy (±s.e.m. of three replicates) is normalized first to total H3 ChIP and then to vector-transduced cells. Light grey bars, vector-transduced cells; dark grey bars, hTERT-transduced cells. *P<0.012; **P<0.006. (d) Analysis of histone marks within the telomeric luciferase gene in response to SIRT6 depletion in hTERT-overexpressing cells. Occupancy is normalized first to total H3 ChIP and then to control siRNA-transfected cells; graph shows mean of four independent knockdown and ChIP experiments, ±s.e.m. Light grey bars, control siRNA-transfected cells; dark grey bars, cells transfected with si SIRT6 no. 1. *P<0.05; **P<0.01 (for individual loci; combining relative occupancy values for all loci,P-values areP=2×10−5andP=2×10−8for H3K9Ac and H3K9me3, respectively).P-value for H3K9Ac at locus A=0.070. Forb–d, labels A–D represent individual loci (within the luciferase gene) assayed by RT–PCR. Forb, andc,P-values were calculated by comparing hTERT-overexpressing cells to vector-transduced cells, using a one-tailedt-test. Ford,P-values were calculated by comparing si SIRT6-transfected cells to control-transfected cells, using a one-tailedt-test. As shown in Figure 4b , telomere elongation (following telomerase overexpression, see Fig. 1b ) led to an increase in the density of total histone H3 near telomeres, suggesting that the silencing effect exerted by long telomeres is due to the formation of a closed telomeric chromatin structure. Consistent with this model, hTERT overexpression led to a marked decrease in H3K9Ac and a significant increase in H3K9me3 at these loci ( Fig. 4c ). Together, these data demonstrate a profound effect of telomere length on telomere-proximal chromatin structure, consistent with previous observations linking TPE to telomere length in yeast [9] , [10] . Notably, a recent report suggests that, in contrast to the well characterized heterochromatic features of long murine telomeres [29] , the shorter telomeres of primary human cells may not be particularly enriched in marks of heterochromatin [30] . Our observation that long telomeres are associated with a more closed chromatin structure may help explain these differences. Figure 4: Characterization of telomere-proximal chromatin changes triggered by telomere elongation and SIRT6 depletion. ( a ) Schematic of the luciferase cassette and real-time PCR primers used in ChIP experiments in b – d . The palindromic nature of the promoter region of the integrated luciferase plasmid precluded the use of primers upstream of the luciferase gene. CEN, centromere. ( b ) Analysis of total H3 occupancy within the telomeric luciferase gene in response to telomere elongation. Data are representative of at least two independent experiments. Light grey bars, vector-transduced cells; dark grey bars, hTERT-transduced cells. ( c ) Analysis of histone marks within the telomeric luciferase gene in response to telomere elongation. Occupancy (±s.e.m. of three replicates) is normalized first to total H3 ChIP and then to vector-transduced cells. Light grey bars, vector-transduced cells; dark grey bars, hTERT-transduced cells. * P <0.012; ** P <0.006. ( d ) Analysis of histone marks within the telomeric luciferase gene in response to SIRT6 depletion in hTERT-overexpressing cells. Occupancy is normalized first to total H3 ChIP and then to control siRNA-transfected cells; graph shows mean of four independent knockdown and ChIP experiments, ±s.e.m. Light grey bars, control siRNA-transfected cells; dark grey bars, cells transfected with si SIRT6 no. 1. * P <0.05; ** P <0.01 (for individual loci; combining relative occupancy values for all loci, P -values are P =2×10 −5 and P =2×10 −8 for H3K9Ac and H3K9me3, respectively). P -value for H3K9Ac at locus A=0.070. For b – d , labels A–D represent individual loci (within the luciferase gene) assayed by RT–PCR. For b , and c , P -values were calculated by comparing hTERT-overexpressing cells to vector-transduced cells, using a one-tailed t -test. For d , P -values were calculated by comparing si SIRT6-transfected cells to control-transfected cells, using a one-tailed t -test. Full size image We next asked whether the reactivation of telomeric luciferase expression resulting from SIRT6 depletion is associated with aberrant loss of heterochromatic marks. Indeed, ChIP assays revealed an increase in the active H3K9Ac mark and loss of the heterochromatic H3K9me3 mark at the telomeric luciferase gene in response to RNAi-mediated SIRT6 depletion ( Fig. 4d ). Thus, SIRT6 is important for generating a proper telomeric chromatin structure that is required for silencing nearby genes. Silencing of a natural telomere-proximal gene requires SIRT6 To date, most studies examining regulators of TPE in yeast and human cells have used integrated reporter genes rather than natural telomere-proximal genes. Thus, little is known about how telomeric silencing regulates endogenous gene expression in human cells. A previously reported screen identified one telomere-proximal human gene—interferon-stimulated gene 15 ( ISG15 ), located ∼ 1 megabase from the telomere—as being regulated by telomere length in primary and cancer cell lines with natural and manipulated telomere lengths [31] . Consistent with this finding, we observed that in our HeLa cell system, telomere lengthening (via expression of ectopic hTERT, Fig. 1b ) led to a reduction in ISG15 messenger RNA levels ( Fig. 5a ). 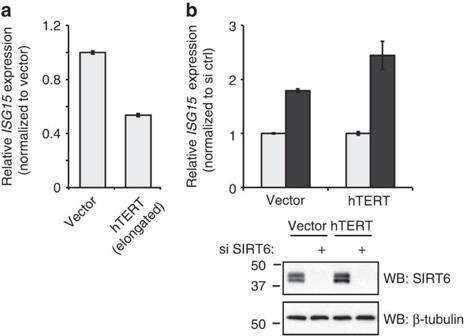Figure 5: Effect of SIRT6 depletion on expression ofISG15, an endogenous telomere-proximal gene. (a)ISG15mRNA levels in vector- and hTERT-transduced HeLa cells were determined by reverse transcription and quantitative real-time PCR and normalized first to β-actin levels and then to vector-transduced cells. (b)ISG15mRNA levels in HeLa cells transfected with control siRNA or si SIRT6 no. 1 were determined as in (a) and normalized first to β-actin and then to control siRNA-transfected cells. Light grey bars, si ctrl; dark grey bars, si SIRT6. Data show the average of three replicates ±s.e.m., and are representative of three independent experiments. Figure 5: Effect of SIRT6 depletion on expression of ISG15 , an endogenous telomere-proximal gene. ( a ) ISG15 mRNA levels in vector- and hTERT-transduced HeLa cells were determined by reverse transcription and quantitative real-time PCR and normalized first to β-actin levels and then to vector-transduced cells. ( b ) ISG15 mRNA levels in HeLa cells transfected with control siRNA or si SIRT6 no. 1 were determined as in ( a ) and normalized first to β-actin and then to control siRNA-transfected cells. Light grey bars, si ctrl; dark grey bars, si SIRT6. Data show the average of three replicates ±s.e.m., and are representative of three independent experiments. Full size image To determine whether SIRT6 is required for TPE-mediated silencing of ISG15 , we assessed ISG15 expression in cells depleted of SIRT6. Strikingly, transient siRNA-mediated depletion of SIRT6 led to an increase in ISG15 expression ( Fig. 5b ), mirroring the results observed with the telomeric luciferase reporter ( Fig. 2a,b ). This result identifies SIRT6 as the first chromatin regulatory protein required for efficient silencing of an endogenous telomere-proximal gene. Here we have reported a new role for SIRT6 in regulating the silencing of genes near telomeres and maintaining the heterochromatic features of telomeric chromatin in human cells. We demonstrate that RNAi-mediated depletion of SIRT6 leads to de-repression of a telomeric transgene, and that recovery of SIRT6 expression is sufficient to re-establish silencing of this transgene. Mechanistically, we find that depletion of SIRT6 disrupts the closed chromatin environment near telomeres. Importantly, we show that SIRT6 is required for repression of an endogenous telomere-proximal gene, suggesting a key role for SIRT6 in maintaining a silencing-competent chromatin structure at natural telomeres. These findings provide the first demonstration of a role for SIRT6 in maintaining transcriptionally silent chromatin domains and identify SIRT6 as the first histone-modifying enzyme that regulates TPE in human cells, thus establishing a new link between SIRT6 and an important ageing-associated molecular phenomenon. Sir2-mediated deacetylation of sub-telomeric histones is important in regulating ageing in S. cerevisiae [6] , and localized changes in telomeric chromatin in late-passage human cells have been linked to cellular senescence [30] . Additionally, telomere shortening has been shown to correlate with degenerative pathologies and shortened health span in mammals [32] , and aberrant expression of silent chromatin has been linked to ageing and cancer [33] , [34] . Because telomeres shorten with each cell division in most somatic human cells, it is possible that telomere erosion—and consequent de-repression of telomere-proximal genes—may in part account for ageing-related changes in gene expression [10] , [35] . In addition, loss of silencing factors from shortening telomeres might lead to a relocalization of these factors from telomeres to other genomic loci, triggering aberrant silencing of non-telomeric genes [36] . By linking SIRT6 to chromatin silencing at telomeres, our findings highlight an evolutionarily conserved role for sirtuin proteins in the silencing of telomere-proximal genes and suggest a role for SIRT6 in modulating ageing-associated changes in chromatin structure and gene expression. Cell culture and transfection HeLa cells harbouring telomeric and internal luciferase transgenes have been previously described [11] . Cell lines 97 (telomeric) and 111 (internal) were used for all experiments except those in Figure 2b , which were performed with cell lines 73 (telomeric) and 115 (internal). siRNA transfections were performed using Dharmafect reagent 1 (Dharmacon), according to the manufacturer's instructions, and cells were collected for luciferase assays and western blots ∼ 72 h post-transfection, unless otherwise indicated. siRNA target sequences are as follows: si SIRT6 no. 1: AAGAATGTGCCAAGTGTAAGA; si SIRT6 no. 2: CCGGCTCTGCACCGTGGCTAA; si SIRT1: GATTTAGACGTGTCCGAAT. Luciferase assays Luciferase assays were performed using the Luciferase Assay Kit (Promega), using 10 μg of lysate and according to the manufacturer's instructions. Each graph represents three biological replicates. Antibodies The antibodies used were as follows: anti-SIRT6 (ref. 37 , 0.4 μg ml −1 ), anti-SIRT1 (Santa Cruz, 0.1 μg ml −1 ), anti-β-tubulin (Millipore, 0.2 μg ml −1 ), anti-H3K9Ac (Sigma, 1.2 μg per ChIP), anti-H3K9me3 (Abcam, 1.2 μg per ChIP), anti-H3 (Abcam, 1.2 μg per ChIP), anti-TRF2 (Imgenex, 5 μg ml −1 ), anti-γ-H2AX (Cell Signaling, 1:400). Chromatin immunoprecipitation and quantitative real-time PCR For chromatin immunoprecipitation (ChIP) [16] , cells were crosslinked with 1% formaldehyde at room temperature for 10–15 min and quenched with 125 mM glycine. Cells were then resuspended in swelling buffer (5 mM Tris–HCl pH 8.0, 85 mM KCl, 1% Nonidet P-40, complete protease inhibitor cocktail (Roche)) for 20 min on ice. Isolated nuclei were resuspended in nuclei lysis buffer (50 mM Tris–HCl pH 8.0, 10 mM EDTA, 1% SDS) and sonicated with a BioRuptor Sonicator (Diagenode). Samples were immunoprecipitated overnight with the indicated antibodies. Immunoprecipitates were captured using nProteinA sepharose (GE Healthcare), washed twice with dialysis buffer (50 mM Tris–HCl pH 8.0, 2 mM EDTA, 0.2% sarkosyl) and four times with IP wash buffer (100 mM Tris–HCl pH 8.5, 500 mM LiCl, 1% Nonidet P-40, 1% deoxycholate), and eluted in elution buffer B (50 mM Tris 8, 200 mM NaCl, 1% SDS, 5 μg ml −1 proteinase K). Following crosslink reversal, ChIP-associated sequences were detected by quantitative real-time PCR using SYBR green and the ABI Prism 7300 sequence detection system (Applied Biosystems). PCR primers depicted in Figure 4 are as follows (forward/reverse, (distance from luciferase ATG in nucleotides)): A: GCACATATCGAGGTGAACATCAC/GCCAACCGAACGGACATTT (133–191); B: GCCCGCGAACGACATTTAT/ACGGTAGGCTGCGAAATGTT (309–374); C: GATCGTGACAAAACAATTGCAC/GGGCCACACCCTTAGGTAAC (559–628); D: AGAGATCCTATTTTTGGCAATCAAA/CGTGATGGAATGGAACAACACT (667–736). For histone mark ChIPs, occupancy values were normalized to total histone H3. Real-time PCR gene expression analysis RNA was extracted from cells ∼ 72 h after siRNA transfection using the RNeasy kit (Qiagen) and reverse transcribed using SuperScript III (Invitrogen) and oligo(dT) primers, according to the manufacturers' instructions. Quantitative real-time PCR analysis was performed on a Roche LightCycler 480 using the manufacturer's Universal Probe Library (UPL) system. Intron-spanning PCR primers are as follows (forward/reverse, (UPL probe number)): ISG15 : TTTGCCAGTACAGGAGCTTG/AGCATCTTCACCGTCAGGTC (no. 76); β-actin: CCAACCGCGAGAAGATGA/CCAGAGGCGTACAGGGATAG (no. 64). Terminal restriction fragment assay For telomere length determination, genomic DNA was purified using the Qiagen DNeasy Blood and Tissue Kit, according to the manufacturer's instructions. 2.5 μg of Rsa I/ Hinf I-digested genomic DNA was separated on a 0.7% agarose TAE gel, transferred to Hybond N+ (GE Healthcare), and detected using a digoxigenin (DIG)-labelled telomere probe, using the TeloTAGGG Telomere Length Assay Kit (Roche). Immunofluorescence For detection of telomere dysfunction-induced foci (TIFs) ∼ 72 h after siRNA transfection, cells seeded on coverslips were permeabilized with Triton X-100 buffer (0.5% Triton X-100, 20 mM Hepes-KOH pH 7.9, 50 mM NaCl, 3 mM MgCl 2 , 300 mM sucrose) for 5–10 min at 4 °C to remove soluble nucleoplasmic proteins. After permeabilization cells were fixed in 3% paraformaldehyde/2% sucrose in PBS for 15 min at room temperature, re-permeabilized in Triton X-100 buffer, and blocked in PBS+1% bovine serum albumin. TIFs were detected using antibodies against TRF2 (Imgenex clone 4A794, 5 μg ml −1 ) and γ-H2AX (Cell Signaling rabbit monoclonal clone 20E3, 1:400) and AlexaFluors 488 and 555, respectively (Invitrogen). Coverslips were mounted using ProLong Gold Antifade reagent with DAPI (Invitrogen) and imaged using a Leica DM5000 B microscope, QImaging Retiga EXi Fast 1394 camera, and QImaging QCapture Pro imaging software. Telomere FISH ∼ 72 h after siRNA transfection, metaphase spreads were prepared by treating cells with 100 ng ml −1 Karyomax colcemid (Invitrogen) for 2.5 h, swelling in 75 mM KCl, and fixing in 3:1 methanol:acetic acid. Telomere fluorescence in situ hybridization (FISH) was performed [16] using the Telomere PNA FISH Kit/Cy3 (Dako), according to the manufacturer's instructions. Slides were mounted using ProLong Gold Antifade reagent with DAPI (Invitrogen) and imaged as described above. How to cite this article: Tennen, R. I. et al . SIRT6 is required for maintenance of telomere position effect in human cells. Nat. Commun. 2:433 doi: 10.1038/ncomms1443 (2011).